Reply to “Quality control requirements for the correct annotation of lipidomics data” 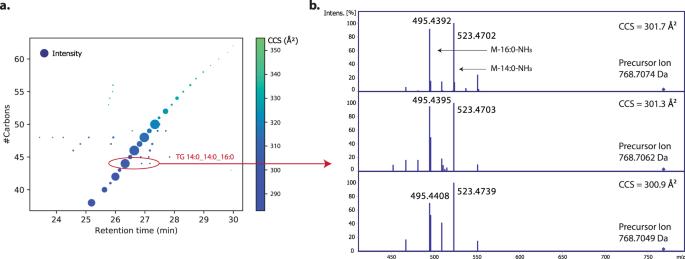Fig. 1: Retention time analysis of triacylglycerols (TGs) with 0 double bonds. aRetention time versus the number of fatty acyl carbons. Dot size indicates the relative ion intensity and dot color visualizes the collisional cross section (CCS).bExperimental MS/MS spectra of the three features highlighted in panel a supporting the annotation of TG14:0_14:0_16:0. 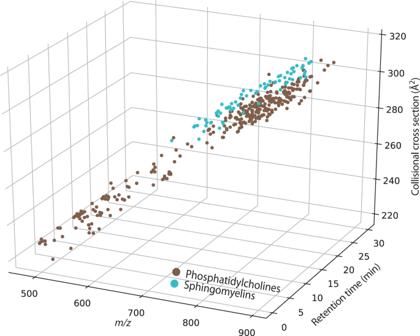Fig. 2: Lipid detection in nanoflow LC-TIMS-MS experiments. Separation of features in a human plasma extract annotated as phosphatidylcholine (PC) and sphingomyelin (SM) lipids inm/z, retention time, and ion mobility dimensions. One outlier is not shown because its CCS value is out of bounds. Further information on research design is available in the Nature Research Reporting Summary linked to this article.